Redox-responsive branched-bottlebrush polymers forin vivoMRI and fluorescence imaging Stimuli-responsive multimodality imaging agents have broad potential in medical diagnostics. Herein, we report the development of a new class of branched-bottlebrush polymer dual-modality organic radical contrast agents—ORCAFluors—for combined magnetic resonance and near-infrared fluorescence imaging in vivo . These nitroxide radical-based nanostructures have longitudinal and transverse relaxation times that are on par with commonly used heavy-metal-based magnetic resonance imaging (MRI) contrast agents. Furthermore, these materials display a unique compensatory redox response: fluorescence is partially quenched by surrounding nitroxides in the native state; exposure to ascorbate or ascorbate/glutathione leads to nitroxide reduction and a concomitant 2- to 3.5-fold increase in fluorescence emission. This behaviour enables correlation of MRI contrast, fluorescence intensity and spin concentration with tissues known to possess high concentrations of ascorbate in mice. Our in vitro and in vivo results, along with our modular synthetic approach, make ORCAFluors a promising new platform for multimodality molecular imaging. Nanoparticle (NP)-based multimodality imaging agents have broad potential for applications in medical diagnostics [1] , [2] , [3] . Of the common modalities, magnetic resonance imaging (MRI) and optical imaging are particularly common in clinical and research laboratories: MRI is used to image millions of patients per year [4] , [5] , while near-infrared (NIR) optical imaging is emerging as a powerful tool for image-guided surgery [6] , and is used routinely to monitor disease progression and nanoparticle biodistribution in animal models [7] , [8] . There are several reports of small molecule [9] , [10] , [11] , [12] , [13] and NP [14] , [15] , [16] , [17] , [18] , [19] , [20] , [21] -based constructs for combined MRI and fluorescence imaging. In some cases, these agents are stimuli-responsive ‘sensors’ that feature enhanced contrast or emission in response to specific cellular signals [22] . For example, Zn(II) [9] , [10] , Cu(II) [11] , [12] , NADH [13] and pH [19] , [20] -responsive dual-modality MRI/fluorescent agents have been designed. Though these systems have provided useful insights into biochemical processes, they are often limited to in vitro imaging studies; the fluorophores used do not absorb/emit in the NIR, which is necessary for in vivo optical imaging. Furthermore, these systems invariably rely on the use of paramagnetic metals to achieve MRI contrast via alteration of the nuclear relaxation times of endogenous protons [23] , [24] . Though widely used in both research and clinical applications, metal-based MRI contrast agents face toxicity concerns [4] , [23] , [25] , [26] ; metal-free MRI/NIR agents could provide a safer alternative for dual-modality in vivo imaging. Recently, Thurecht and coworkers reported a novel hyperbranched polymer NP construct for simultaneous in vivo 19 F-MRI and NIR optical imaging [21] . Though this elegant system avoids metals, it requires the use of 19 F-MRI, which is not yet commonplace in the clinic [14] . Furthermore, though in vitro pH-responsive 19 F imaging agents have very recently been reported [27] , [28] , these systems have not yet been rendered responsive to specific biological molecules for molecular MRI. Thus, to our knowledge, there are no examples of entirely organic, stimuli-responsive, dual-modality MRI/NIR imaging agents for molecular imaging applications. In an effort to design such materials, we were drawn to the unique properties of paramagnetic nitroxides. Nitroxides have been extensively studied as metal-free ‘organic radical contrast agents’ (ORCAs) for MRI [29] , [30] , [31] , [32] . They typically show minimal toxicity [33] , and they are reduced to diamagnetic hydroxylamines at variable rates in response to physiological reducing agents [33] , [34] , [35] . This feature has been exploited for selective MR imaging of redox processes in vivo [36] , [37] , [38] , [39] . The key disadvantages of nitroxides are their low relaxivity compared with metals [31] and their very rapid in vivo reduction (on the order of minutes for most nitroxides) [36] , [37] , [38] , [39] . Nanostructured ORCAs that carry multiple reduction-resistant nitroxides can potentially overcome these limitations [31] , [32] , [40] , [41] , [42] . Nitroxides are also well known for their ability to quench excited singlet states through catalysis of intersystem crossing [43] , [44] . This property has been exploited for the development of nitroxide-fluorophore conjugates, where emission from the fluorophore is enhanced upon nitroxide reduction. Such molecules have been used for imaging redox processes in vitro [45] , [46] , [47] , [48] , [49] and for analysis of oxidation-induced polymer degradation [50] , [51] . We report here redox-responsive branched-bottlebrush copolymer NPs (ORCAFluors) that possesses a high nitroxide density for MRI and an NIR fluorophore for optical imaging. Compared with other nitroxide-based MRI agents, ORCAFluors show excellent stability towards biological reducing agents and substantial in vitro and in vivo MRI contrast. Furthermore, ORCAFluors display compensatory redox behaviour whereby ascorbate-induced nitroxide reduction leads to the loss of MRI signal and enhanced fluorescence emission. To the best of our knowledge, ORCAFluors represent the first entirely organic dual-modality imaging system that is suitable for molecular imaging of redox processes in vivo using both MRI and NIR optical imaging. Synthetic strategy Our ORCAFluor design is based on the branched-bottlebrush polymer architecture [52] , [53] . Branched-bottlebrush polymers are nanoscopic copolymers with two or more distinct functional domains, at least one of which is a polymer, grafted to every repeat unit of a polymer backbone. Such polymers can be readily synthesized via Ru-initiated graft-through ring-opening metathesis polymerization (ROMP) [54] of norbornene-terminated branched macromonomers (MMs). The final size and composition of the polymer depends on the size and composition of the MM, as well as the ratio of MM to ROMP initiator. For this study, we designed two novel poly(ethylene glycol) (PEG)-based MMs (see Supplementary Methods for synthetic details): one carries a reduction-resistant spirocyclohexyl nitroxide (chex-MM 1, Fig. 1a ) that provides in vivo MRI contrast enhancement [31] , [55] ; the other carries Cy5.5 for NIR fluorescence imaging (Cy5.5-MM 2, Fig. 1a ). PEG is included in both the structures to increase the hydrophilicity of the final NP and provide for extended circulation in vivo [56] . The structure of each MM was confirmed by matrix-assisted laser desorption/ionization mass spectrometry ( Supplementary Fig. 1 ) and NMR spectroscopy. 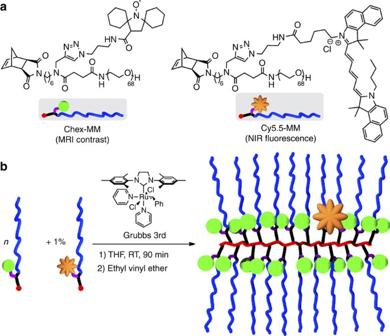Figure 1: ORCAFluor precursors and synthetic scheme. (a) Structures of branched macromonomers (MMs) used in this study. (b) General procedure for the graft-through ROMP synthesis of ORCAFluor imaging agents. RT, room temperature; THF, tetrahydrofuran. Figure 1: ORCAFluor precursors and synthetic scheme. ( a ) Structures of branched macromonomers (MMs) used in this study. ( b ) General procedure for the graft-through ROMP synthesis of ORCAFluor imaging agents. RT, room temperature; THF, tetrahydrofuran. Full size image We first tested the ROMP of chex-MM in the absence of Cy5.5-MM. A series of nitroxide-loaded bottlebrush polymers were prepared via exposure of chex-MM to Grubbs 3rd generation initiator for 90 min ( Fig. 1b ). After this time, the reactions were quenched with excess ethyl vinyl ether. Gel permeation chromatography ( Supplementary Fig. 2 ) analysis of the crude polymerization reactions indicated that the MM conversion was greater than 95% for all n values from 13 to 141. These results agree with our previous observations in related nitroxide-labelled ROMP polymer systems [53] , [57] , [58] ; the graft-through ROMP process is extremely efficient. For this range of n values, we expect the particles to display a spherical, star-like solution structure. Dynamic light scattering analysis revealed hydrodynamic diameters ( Supplementary Table 1 ) that ranged from 13 to 24 nm as n varied from 13 to 141, respectively. This range is suitable for systemic in vivo administration; PEGylated particles of this size display enhanced circulation times in blood and selective tumour uptake via the enhanced permeation and retention effect [59] . Characterization of nitroxide-functionalized branched-bottlebrush polymers Electron paramagnetic resonance (EPR) spectroscopy was used to characterize the spin environment and concentration in these polymers. As expected for the branched-bottlebrush polymer architecture with a high nitroxide density near the poly(norbornene) backbone [53] (for example, P1 with n =54), the EPR spectrum is significantly broader than that of chex-MM ( Fig. 2a ). The spin concentrations for all the polymer samples were typically >90%. 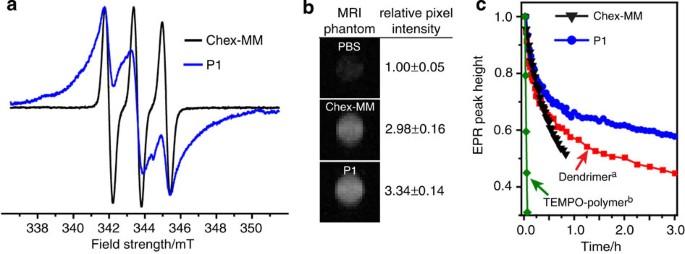Figure 2: Properties of nitroxide-loaded branched-bottlebrush polymers. (a) EPR spectra of chex-MM compared withn=54 bottlebrush polymer P1. (b) MRI phantoms and relative contrast enhancements (compared with PBS buffer) of chex-MM and P1. (c) Analysis of nitroxide reduction in response to ascorbate.a‘dendrimer’ referes to previously reported fourth generation spirocyclohexyl nitroxide-functionalized poly(propyleneimine) dendrimer31.b‘TEMPO-polymer’ refers to previously reported 2,2,6,6-tetramethyl-1-piperidinyloxy (TEMPO)-functionalized branched-bottlebrush polymers53. Figure 2: Properties of nitroxide-loaded branched-bottlebrush polymers. ( a ) EPR spectra of chex-MM compared with n =54 bottlebrush polymer P1. ( b ) MRI phantoms and relative contrast enhancements (compared with PBS buffer) of chex-MM and P1. ( c ) Analysis of nitroxide reduction in response to ascorbate. a ‘dendrimer’ referes to previously reported fourth generation spirocyclohexyl nitroxide-functionalized poly(propyleneimine) dendrimer [31] . b ‘TEMPO-polymer’ refers to previously reported 2,2,6,6-tetramethyl-1-piperidinyloxy (TEMPO)-functionalized branched-bottlebrush polymers [53] . Full size image Longitudinal ( r 1 ) and transverse ( r 2 ) relaxivities for chex-MM and this series of branched-bottlebrush polymers were measured using a Bruker 7T MRI instrument ( Supplementary Table 1 , Supplementary Fig. 3 ). The r 1 and r 2 values for chex-MM were 0.21 mM −1 s −1 and 0.30 mM −1 s −1 , respectively. As expected for slowly diffusing NPs [5] , [24] , the branched brush polymers displayed increased relaxivity values ( Supplementary Table 1 ). For example, the values for P1 were r 1 =0.32 mM −1 s −1 and r 2 =0.82 mM −1 s −1 , which correspond to 52 and 173% increases, respectively. The molecular relaxivities of P1 can be obtained by multiplying the per nitroxide values by the average number of nitroxides per particle: r 1mol =15.7 and r 2mol =40.3 for P1. These values are comparable to clinically used metal-based contrast agents [23] ; we reasoned they would provide sufficient contrast for in vivo imaging applications. A T 1 -weighted MRI phantom for P1 (10 mM nitroxide in phosphate-buffered saline (PBS)) shows a 3.34±0.14-fold enhancement compared with PBS alone ( Fig. 2b ). These relative enhancements are in qualitative agreement with the r 1 values, the T 1 and T 2 1 H relaxation times and the parameters used to obtain the phantom images. Next, we assessed the nitroxide reduction kinetics of these materials in the presence of ascorbate. Ascorbate is known to be a major contributor to nitroxide reduction in vivo where concentrations range from micro- to millimolar depending on the tissue type [34] , [60] , [61] . This reduction is very rapid for most nitroxide derivatives; we hypothesized that the combination of the known reduction-resistant spirocyclohexyl nitroxide with the sterically shielded branched-bottlebrush architecture would provide enhanced reduction resistance and extend the utility of these materials in vivo . The reduction of chex-MM and P1 in response to ascorbate (20 equivalents (equiv.) per nitroxide) was monitored by EPR spectroscopy ( Fig. 2c ). The quenching results were compared with an analogous 2,2,6,6-tetramethyl-1-piperidinyloxy (TEMPO)-conjugated branched-bottlebrush polymer [53] ( Fig. 2c , green) and a spirocyclohexyl nitroxide-conjugated poly(propylenimine) (PPI) dendrimer ( Fig. 2c , red) [31] . As expected, the TEMPO-polymer was reduced very rapidly under these conditions ( Fig. 2c , green). The macromonomer ( Fig. 2c , black) and dendrimer ( Fig. 2c , red) showed increased reduction resistance due to the spirocyclohexyl nitroxide and the addition of PEG. The branched-bottlebrush polymer P1, with spirocyclohexyl nitroxides shielded by PEG at every monomer unit, was the least susceptible to reduction ( Fig. 2c , blue). These results support our hypothesis that the combination of the branched-bottlebrush architecture with the reduction-resistant spirocyclohexyl nitroxide will enhance reduction resistance. Note that similar initial rate constants for reduction of nitroxides were obtained using ascorbate/glutathione ( Supplementary Table 2 ). ORCAFlour synthesis and in vitro analysis Encouraged by these results with P1, we prepared an analogous ORCAFluor (OF1) via copolymerization of 55 equiv. of chex-MM and 1% (0.55 equiv.) Cy5.5-MM ( Fig. 1 ). We reasoned that this approach would provide a sufficient amount of Cy5.5 for fluorescence imaging with minimal impact on nitroxide density and MRI contrast. GPC analysis of OF1 ( Supplementary Fig. 4 ) shows a monomodal molar mass distribution with >99% MM conversion. The refractive index and 675 nm absorption traces overlap, which suggests that Cy5.5 is successfully incorporated into the polymer. Cryogenic transmission electron microscopy imaging of OF1 revealed a spherical morphology with an average diameter of 19±8 nm ( Supplementary Fig. 5 ); this value agrees closely with the hydrodynamic diameter for P1 as measured by dynamic light scattering. We reasoned that the dense nitroxide backbone of OF1 would quench the Cy5.5 emission ( Fig. 3a ); nitroxide reduction would then lead to decreased MRI contrast and an enhanced fluorescence signal. Fluorimetric analysis ( Supplementary Figs 6 and 7 ) of OF1 in the absence of ascorbate suggests that Cy5.5 fluorescence is not completely quenched. However, when two different samples of OF1 were treated with 60 equiv. of ascorbate, a rapid ~120% increase in fluorescence was observed ( Fig. 3b , black circles and squares). When 30 equiv. ( Fig. 3b , black triangles) or 10 equiv. ( Fig. 3b , white triangle) were added to OF1, the emission intensity increased by ~80% and ~25%, respectively. Addition of another 30 equiv. or 50 equiv., respectively, to these samples increased the emission to the same point as the 60 equiv. sample. The average total emission increase was 119±5% for this series of experiments. When a control polymer with 1% Cy5.5 and no nitroxides was exposed to 60 equiv. of ascorbate, no significant increase in emission intensity was observed ( Fig. 3b , grey circles). Furthermore, OF1 showed no significant response to the reducing agent glutathione (GSH) alone; addition of ascorbate to a mixture of OF1 and GSH led to a 250% increase in fluorescence intensity ( Fig. 3b , white circles). GSH is known to enhance the overall extent of ascorbate-mediated nitroxide quenching via reduction of ascorbate radicals that can otherwise re-oxidize newly formed hydroxylamines [35] , [62] . Collectively, these results strongly suggest that fluorescence enhancement of OF1 occurs selectively in response to ascorbate-induced nitroxide reduction. Though this enhancement is not as large as observed for small-molecule sensors where the nitroxide is directly coupled to a fluorophore [44] , [49] , we were encouraged to explore the potential of OF1 for in vivo dual-modality imaging (vide infra). 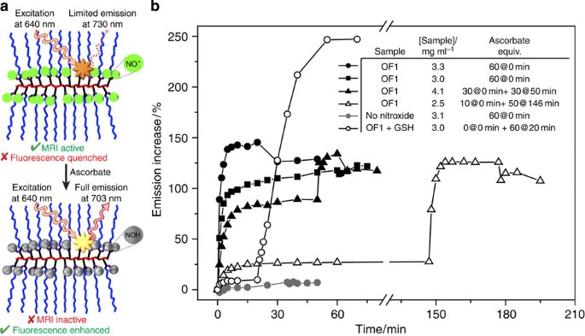Figure 3: Redox-sensitive dual-modality imaging mechanism. (a) Schematic for dual-modality molecular imaging in response to nitroxide reduction. (b) Emission behaviour of OF1 and a control polymer with Cy5.5 and no nitroxides upon exposure to varied amounts of ascorbate or glutathione (GSH) in PBS buffer. The solution pH before and after addition of 60 equiv. ascorbic acid was 7.0 and 6.31, respectively; this pH change has no affect on Cy5.5 absorbance/emission. equiv., equivalent. Figure 3: Redox-sensitive dual-modality imaging mechanism. ( a ) Schematic for dual-modality molecular imaging in response to nitroxide reduction. ( b ) Emission behaviour of OF1 and a control polymer with Cy5.5 and no nitroxides upon exposure to varied amounts of ascorbate or glutathione (GSH) in PBS buffer. The solution pH before and after addition of 60 equiv. ascorbic acid was 7.0 and 6.31, respectively; this pH change has no affect on Cy5.5 absorbance/emission. equiv., equivalent. Full size image Before imaging studies, we sought to assess the preliminary toxicity and pharmacokinetic properties of OF1. PEGylated ROMP nanostructures typically display low toxicity and extended circulation time in vivo [63] , [64] , [65] . We hypothesized that OF1, which possess a dense PEG corona, would behave similarly. In v itro , no discernible toxicity was observed as determined by cell viability assays with HeLa cells (ATCC, Supplementary Fig. 8 ). Little gross toxicity was observed in healthy BALB/c mice intravenously administered OF1 doses from 1 to 40 mg per mouse (0.04–2 g kg −1 ); acceptable [66] , [67] (1–10%) body weight decreases over the first 5 days after injection were followed by a return to the initial body weight within 10 days ( Supplementary Fig. 9 ) and no apparent behavioural changes. Preliminary pharmacokinetics data were obtained via fluorescence imaging (IVIS, Cy5.5 λ ex / λ em =640/700 nm, Xenogen) of blood samples taken at various time points after an injection of 30 mg of OF1. An initial rapid clearance was observed (~60% over 30 min), which was followed by a slow linear decay from 40 to 20% over 3 days ( Supplementary Fig. 10 ). Note that these values are based on comparison to the % of injected fluorescence, which is complicated by nitroxide reduction in the blood (vide infra). Nevertheless, the data indicate that a significant fraction of the particle is present in the blood even after 3 days. This extended circulation suggests that OF1 could be used in the future for tumour-targeted imaging via the enhanced permeation and retention effect [59] . In an effort to demonstrate the dual-modality imaging potential of OF1, four NCR nude mice were anaesthetized with 1–2% isofluorane and imaged via IVIS and T 1 -weighted MRI (see Supplementary Methods for details). The mice were then systemically administered (tail vein) 30 mg of OF1 dissolved in pH 7.4 PBS solution. After 30 min, the mice were anaesthetized and imaged by MRI and IVIS. At this point, a blood sample was taken, the mice were killed (CO 2 chamber), and organs were collected, imaged with IVIS and frozen on dry ice. 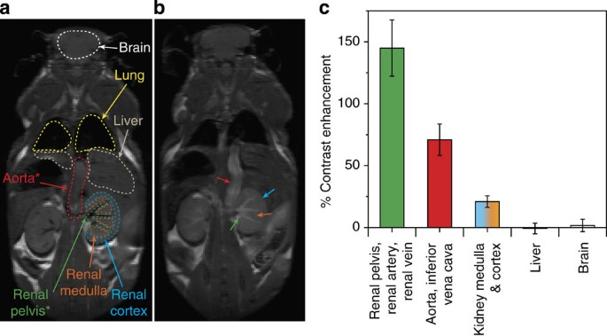Figure 4: MRI imaging studies. (a) MR image of whole mouse before OF1 injection with specific organs/tissues outlined for reference. Red asterisk: structure labeled as aorta could also include inferior vena cava. Green asterisk: structure labeled renal pelvis could also include renal artery and renal vein. (b) MR image of the same mouse 30 min after OF1 injection. (c) Quantitative analysis (mean±s.e.) of volume-average MR image contrast enhancement for four mice 30 min after OF1 injection. The values correlate with [spin] values obtained by EPR (videFig. 6). Figure 4a,b show pre- and 30 min post-OF1 injection MRI images, respectively. Values of volume-averaged % contrast enhancement ( Fig. 4c ) were obtained from region of interest (ROI) analysis using ImageJ software. The largest contrast enhancements (145±23% and 71±13%) were observed in the regions associated with the renal pelvis, renal artery, renal vein (labeled green in Fig. 4a,b ) and the aorta (labeled red in Fig. 4a,b ), respectively. These data suggest a high concentration of non-reduced OF1 in the blood, which agrees well with the pharmacokinetic data discussed above ( Supplementary Fig. 10 ). These enhancements are comparable with the highest reported for entirely organic MRI contrast agents [31] , [32] . Figure 4: MRI imaging studies. ( a ) MR image of whole mouse before OF1 injection with specific organs/tissues outlined for reference. Red asterisk: structure labeled as aorta could also include inferior vena cava. Green asterisk: structure labeled renal pelvis could also include renal artery and renal vein. ( b ) MR image of the same mouse 30 min after OF1 injection. ( c ) Quantitative analysis (mean±s.e.) of volume-average MR image contrast enhancement for four mice 30 min after OF1 injection. The values correlate with [spin] values obtained by EPR (vide Fig. 6 ). Full size image The renal medulla and cortex showed a small contrast increase (21±5%), while the brain and the liver showed no detectable enhancement. We were particularly surprised by the latter result, given that nanoparticles similar in size to OF1 are known to accumulate in the liver [56] . Unlike humans, mice possess the requisite enzyme, gulonolactone oxidase, for ascorbate biosynthesis; this process occurs in the liver, where the ascorbate concentration is in the mM regime [68] , [69] . Thus, we suspected that ascorbate-induced nitroxide reduction in the liver could explain the low MRI contrast in this organ. If so, a strong fluorescence signal should be observed in the liver. 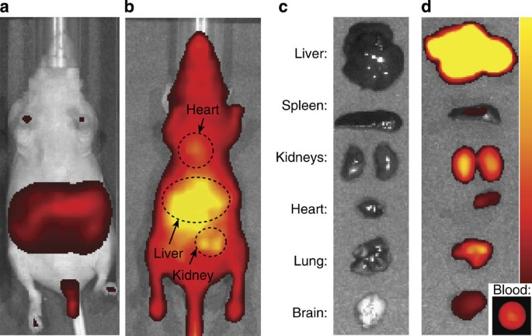Figure 5: NIR fluorescence imaging studies. (a) IVIS image of whole mouse before OF1 injection. (b) IVIS image of the same mouse ina30 min after OF1 injection. (c)Ex vivoIVIS images of organs before OF1 injection. (d)Ex vivoIVIS images of organs and blood sample after OF1 injection. Figure 5 shows whole-animal fluorescence and ex vivo necropsy IVIS images for the same animal imaged via MRI above. Minimal autofluorescence is observed before OF1 injection ( Fig. 5a ); 30 min after injection, the maximum fluorescence is observed in the liver and kidneys with a small amount of fluorescence observable in the heart ( Fig. 5b ). These results are corroborated by tissue necropsy data ( Fig. 5c,d ), which shows the greatest fluorescence intensity in the liver and kidneys. We also observed significant fluorescence in the blood ( Fig. 5d ) and lung, the latter of which is saturated with blood. This strong signal in the blood, which coincides with the regions of greatest MRI contrast, suggests that the particle is indeed present in the blood mostly in a non-reduced state. The observation of maximal fluorescence in the liver supports our hypothesis that OF1 accumulates in the liver, but that the nitroxides are more reduced in this organ. Figure 5: NIR fluorescence imaging studies. ( a ) IVIS image of whole mouse before OF1 injection. ( b ) IVIS image of the same mouse in a 30 min after OF1 injection. ( c ) Ex vivo IVIS images of organs before OF1 injection. ( d ) Ex vivo IVIS images of organs and blood sample after OF1 injection. Full size image To further support these results, EPR spectra of tissue homogenates were obtained for two sets of mice killed 30 min and 24 h after OF1 injection ( Fig. 6a , Supplementary Fig. 11 ); these data were used to correlate the spin concentration (that is, % injected dose of nitroxide per gram of tissue) with fluorescence (that is, % fluorescence of injected dose per gram of tissue) as a function of tissue type and time after injection ( Fig. 6b ). Statistically significant decreases in spin concentration ([spin]) were observed between the 30 min and 24 h time points for all organs studied, however, 5.6±0.7% of the injected spin dose remained in the blood, whereas only 0.3±0.1% remained in the liver where the ascorbate concentration is higher. If a decrease in [spin] were simply due to the changes in biodistribution or excretion of the particle, then we would expect a concomitant decrease in fluorescence. For example, the kidney showed a marked decrease in fluorescence after 24 h, which suggests that the particle does not accumulate in the kidney. In contrast, the liver, brain, heart and blood all showed no significant decreases in fluorescence after 24 h, despite the decrease in [spin]. After 24 h, we would expect the concentration of OF1 in the blood to decrease significantly; the observation of a similar fluorescence at 30 min and 24 h is most likely due to fluorescence enhancement in response to nitroxide reduction. Notably, the liver and the brain, where the ascorbate concentration is the greatest [68] , showed the least amount of nitroxide after 24 h (none was detectable in the brain tissue), but a significant amount of fluorescence. Taken together, these results suggest that there is a correlation between ascorbate concentration and OF1 fluorescence, and confirm that the dual-modality nature of OF1 can be used to provide complementary information related to redox processes in vivo. 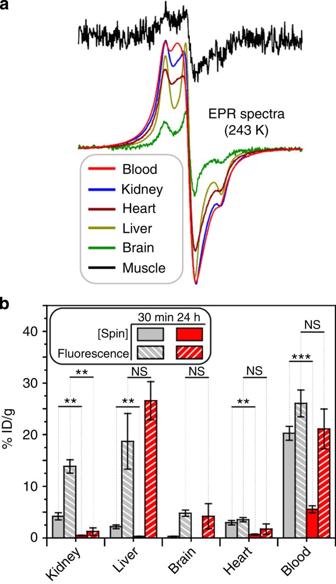Figure 6:Ex vivospin and fluorescence quantification. (a) EPR spectra of blood and homogenized tissue samples. (b) Recovered fluorescence intensity and spin concentration in selected tissues. Error bars represent s.e.m. values obtained from four and three mice at 30 min and 24 h, respectively. Statistical comparisons were made with a student’st-test: **P<0.01 and ***P<0.001. NS, not significant. Figure 6: Ex vivo spin and fluorescence quantification. ( a ) EPR spectra of blood and homogenized tissue samples. ( b ) Recovered fluorescence intensity and spin concentration in selected tissues. Error bars represent s.e.m. values obtained from four and three mice at 30 min and 24 h, respectively. Statistical comparisons were made with a student’s t -test: ** P <0.01 and *** P <0.001. NS, not significant. Full size image In conclusion, we have demonstrated the synthesis, characterization and preliminary in vivo analysis of a new class of entirely organic ascorbate-sensitive dual-modality molecular imaging agents. These new ORCAFluors were prepared using graft-through ROMP reactions of spirocyclohexyl nitroxide and Cy5.5-conjugated MMs. Exposure of ORCAFluor OF1 to ascorbate leads to nitroxide reduction and enhanced fluorescence emission. In vivo studies confirmed that OF1 displayed significant MRI contrast enhancement (among the highest known for organic MRI contrast agents), as well as fluorescence emission that correlates with ascorbate concentration in vitro and in vivo . To our knowledge, this work represents the first example of a responsive organic agent for dual 1 H MRI contrast enhancement and live whole-animal fluorescence imaging. The long in vivo circulation of these particles, and their redox-responsive properties, could make them applicable for tumour imaging studies. Our modular ORCAFluor design and flexible synthetic strategy, which is amenable to incorporation of other functionalities, such as drugs [70] and cellular targeting agents, make these new particles a promising platform for further development as redox-sensitive theranostic agents. General methods Precursor syntheses, reagent information, and in vitro MRI relaxivity quantification are detailed in the Supplementary Methods . Please see Supplementary Fig. 12 for PEG-amine synthesis setup, Supplementary Figs 13–16 for NMR spectra, and Supplementary Table 3 for in vivo spin concentration analysis. Instrumentation information can be found in Supplementary Note 1 . Details of MRI phantom intensity as a function of relaxivity ( Fig. 2b ) are provided in Supplementary Note 2 . General procedure for branched-bottlebrush polymer synthesis by ROMP All ROMP reactions were conducted following the same general procedure. The representative method described below is specific for OF1; polymers with different degrees of polymerization can be readily prepared by varying the macromonomer to initiator ratio. Note: all polymerizations were performed under nitrogen atmosphere. Chex-MM (198 mg, 0.05 mmol) and Cy5.5-MM (2.0 mg in 20 μl, 0.5 μmol) were combined in a 4 ml vial and dissolved in 0.795 ml tetrahydrofuran. A solution of Grubbs 3rd generation bispyridine initiator (0.278 ml of 4 mg ml −1 initiator solution, 1 μmol) was added to the vial and the resulting reddish-brown solution was stirred at room temperature for 90 min. After this time, the reaction was quenched with one drop of ethyl vinyl ether. An aliquot of the reaction solution was taken for GPC analysis; the remainder was transferred to a 15 kDa molecular weight cutoff dialysis tubing (Spectrum Laboratories) with 5 ml of nanopure water. The polymer was dialysed against 500 ml of nanopure water (three rounds of fresh water were added with 2 h intervals between each solvent exchange) with gentle stirring. The polymer solution was then lyophilized to dryness, and stored in the dark at 4 °C. GPC traces for OF1 and other representative polymers prior to dialysis are provided in Supplementary Figs 2 and 4 . Fluorimetric analyses Analysis of Cy5.5 fluorescence in various branched-bottlebrush polymer samples was performed by monitoring excitation and emission at 640 and 703 nm, respectively. Slit widths of 5 nm for excitation and 7 nm for emission were used for all studies. Polymer samples (OF1 or control polymer with no nitroxide) were dissolved in 2 ml of pH 7.4 1X PBS buffer; ultraviolet/visible and fluorescence spectra were collected. Aliquots of ascorbic acid were then added to the cuvette as outlined in Fig. 3b . Emission spectra were repeatedly obtained until no change was observed. A representative series of spectra are shown in Supplementary Fig. 7 . Note: The pH was measured before and after addition of 60 equiv. of ascorbic acid; the values were 7.0 and 6.31, respectively. The absorption/emission properties of Cy5.5 are not pH dependent. Kinetics of nitroxide quenching by EPR spectroscopy The results of kinetic measurements are summarized in Supplementary Table 2 . The ascorbate solution was made with ascorbic acid, sodium phosphates (<30 p.p.m. transition metals), sodium hydroxide and diethylenetriaminepentaacetic acid (DTPA, 0.1% (mol/mol) to sodium phosphates) at pH 7.4. This solution was used to dissolve the powder of reduced L -glutathione (GSH), providing the ascorbate/GSH solution, as needed. Solutions of the agents were prepared in phosphate buffer, which was made from sodium phosphates and DTPA (0.1% (mol/mol) to sodium phosphates) at pH 7.4. The kinetic runs were carried out in the presence of a 250-fold molar excess of sodium phosphates with a 20-fold molar excess of ascorbate (or 20-fold of ascorbate and 10-fold of GSH). Before a typical kinetic run, equal volumes of the freshly prepared solution of ascorbate (or ascorbate/GSH) and the solution of agent were combined, vortexed for a few seconds and then the resultant mixture was drawn into three or four EPR-quality quartz capillary tubes (0.6-mm inner diameter). The capillaries were stoppered with parafilm and placed in a 5-mm outer diameter EPR sample tube in the cavity of X-band spectrometer. The peak height of the low-field line of the triplet was measured as a function of time. Microwave power was kept under 6.5 mW and the temperature was controlled at 295 K with a nitrogen flow system. Phantom relaxivities by MRI Monomers and polymers were transferred as solutions in dichloromethane to a set of accurately weighed clean vials, and then evacuated to a constant mass in Schlenk containers (1 mTorr-vacuum). For selected monomers and polymers, small samples (0.4–0.8 mg) were examined by 1 H NMR spectroscopy in chloroform- d (500 MHz, cryoprobe, 3-mm tubes); only monomer chex-MM had a very small residue of dichloromethane, whereas all the other samples were solvent free. To each vial containing the sample, 0.5 mM PBS (0.800 ml, pH 7.2 checked with pH meter) was added, to provide homogenous-to-turbid stock solutions. Spin concentrations of stock solutions were determined by EPR spectroscopy. Serial dilution (100–10% in 10% increments) of each stock solution provided an array of ten 0.1-ml-samples in PCR tubes; for each T 1 and T 2 measurement of 1 H in water, the array of ten 0.1-ml samples and 0.1-ml sample of buffer (11 PCR tubes) were used. T 1 and T 2 , measured at the University of Nebraska Medical Center, were obtained using coronal T 1 and T 2 map imaging protocols ( Supplementary Table 1 and Supplementary Fig. 3 ). T 1 mapping was done using a progressive saturation RARE T 1 mapping measurement with RARE factor=4, First TE and spacing of 6.4 ms, TR=10,000, 5,000, 3,000, 1,500, 1,200, 800, 500, 450, 400, 350 and 300 ms, 60 mm field of view, 1 mm slice thickness, one slice for a total acquisition time of 10 min. T 2 mapping was done using CPMG-phase-cycled multiecho imaging of all sample concentrations including buffer in a single image. Acquisition parameters were: 10 echo, TE=10 ms, one 1 mm thick slice, 256 × 128 matrix, one average, 3000, ms repetition time, 60 mm field of view, for a total acquisition time of 10 min. T 1 and T 2 values were extracted from each sample in the image using ROIs in the image sequence analysis tool in Paravision 5.1. T 2 values were determined by using the even-numbered echoes, fitting the noise floor using the highest free radical concentration and fixing the value for the remaining samples in each image. Cell culture and in vitro toxicity HeLa cells (ATCC) were maintained in MEM Media supplemented with 1% penicillin/streptomycin and 10% fetal bovine serum in 5% CO 2 humidified atmosphere (37° C). Cells were plated in 96-well plates at 10,000 cells per well and grown for 24 h before treating with varied concentrations of polymer. Each polymer concentration was represented by four replicate wells. After 48 h, the cells were incubated for 4 h with thiazolyl blue tetrazolium bromide (MTT). Reduced thiazoyl tetrazolium formazan was then solubilized with dimethyl sulfoxide, and cell viability was calculated on the basis of the absorbance at 550 nm. Animal usage All procedures involving animals were reviewed and approved by the MIT Committee for Animal Care. Toxicity and pharmacokinetics studies were performed on healthy female BALB/c mice aged 12–16 weeks. MRI studies were performed on healthy female NCR nude mice that received an alfalfa-free diet to minimize autofluorescence. All studies involving animals were performed on groups of n =4 or n =5 to provide statistical significance. Exclusion criteria included human error in NP administration. In vivo toxicity and pharmacokinetics Eight polymer solutions ranging from 0.1–40 mg of OF1 in sterile pH 7.4 PBS buffer were prepared. To find an initial toxicity threshold, each solution was administered to one mouse per particle solution. NP solutions were passed through a 0.2 micron filter before injection via catheter into the tail vein. All of these doses appeared to be well tolerated. Thus, two groups of five animals were dosed with 30 or 40 mg of OF1. Animals receiving 40 mg of OF1 demonstrated higher weight loss and some initial lethargy, while animals receiving 30 mg displayed no adverse physical effects; the 30 mg dosage was used for all subsequent imaging studies. In vivo MRI and IVIS MRI experiments were conducted at the Koch Institute for Integrative Cancer Research at MIT using a Varian 7T/310/ASR-whole mouse MRI system. T 1 -weighted MR images were collected using the fast spin echo multiple slices pulse sequence with minimum repetition time (TR)=739 ms, ESP=9.52 ms, ETL=4, a 256 × 256 matrix and four averages over 18 slices at 1 mm thickness. Scans were collected with respiratory gating (PC-SAM version 6.26 by SA Instruments Inc.) to avoid confounding noise due to chest movement. Respiratory rate and animal temperature were closely monitored during image collection. In vivo fluorescence images were obtained on an IVIS Spectrum bioluminescent and fluorescent imaging system from Xenogen. Excitation and emission values (640 nm, 700 nm, respectively) were kept constant, and exposure times from 2–10 s were used. Epi-fluorescence is reported in radiant efficiency and used only as comparison between pre- and post-injection values. MRI and IVIS images were obtained for each animal ( n =4) before administration of OF1. Mice were fit with tail vein catheters and slowly injected with OF1 solution. Thirty minutes or 24 h after injection was complete, the mice were imaged via both IVIS and MRI, and then immediately killed in a CO 2 chamber for tissue collection and fluorescence imaging (vide infra). Organs were briefly washed with saline to remove any exogenous blood from the dissection process. In vivo MRI and IVIS data analysis ROI around each organ was manually selected for a given image slice. The average intensity and area of the ROI were measured. This procedure was repeated for each image slice where the organ/tissue was visible. Using Excel (Microsoft), the average intensity of each ROI was multiplied by its area. These values were then summed together for all image slices of a given organ. This sum was divided by the sum of the ROI areas for the same organ to provide the volume-averaged intensity. The same procedure was repeated for images of four mice collected before and 30 min after injection of OF1 (eight images total). Volume-averaged intensity increases (shown in Fig. 4c ) were obtained from the following equation: ((contrast 30 min after injection)−(contrast before injection))/(contrast before injection) × 100%. The values for % contrast enhancement were normalized by the muscle, which was assumed to be zero. Note that this normalization changed the final values by <10%. Ex vivo fluorescence methods After collecting in vivo MRI and fluorescence data (vide supra), mice were killed in a CO 2 chamber and immediately dissected to remove the kidneys, liver, spleen, heart, lungs, brain and a section of flank muscle tissue. Organs were quickly washed with PBS buffer to remove excess blood from the necropsy process. Extracted organs were placed on a black, non-emitting background for fluorescence analysis. IVIS parameters were identical to those used for in vivo measurements. Ex vivo EPR spectroscopy The animal tissues were shipped in dry ice from MIT to University of Nebraska in centrifuge tubes. Upon receipt, the tubes were stored in liquid nitrogen. For preparation of EPR samples, the tissues samples were temporarily moved from the liquid nitrogen storage to dry ice. Each tissue sample, one at a time, was rapidly thawed, and then transferred to a weighed vial. Then, 0–500 μl of PBS buffer (0.5 mM, pH=7.2) was added. The sample with PBS was then put into an ice-water bath and homogenized with a rotor stator homogenizer, and then pipetted to a 4-mm outer diameter EPR sample tube. The samples were degassed by sonication, as needed (for example, when gas bubbles were visible). The EPR tube was capped, sealed with parafilm and then stored briefly in acetone-dry ice bath before the measurement of spin concentration. The spin concentrations of nitroxide radicals in tissues (μmol g −1 , μmol of S =½ nitroxide radical per gram of tissue) were measured at −30 °C (243.2 K), to increase signal-to-noise for the aqueous samples. Measurements of the tissue samples were alternated with the measurements of the references for spin concentration (see next paragraph) and g -value (2,2-diphenyl-1-picrylhydrazyl powder was used as a g -value reference). For tissue samples with low signal-to-noise, the cavity background was recorded with identical parameters as for the tissue sample (including identical number of scans and identical receiver gain). Typical parameters were as follows: microwave attenuation (20 dB), modulation amplitude (5 Gauss), spectral width (300 Gauss), resolution (512 points), conversion (40.96), time constant (10.24) and sweep time (20.97 s.); these parameters were kept identical for the tissues, references and cavity backgrounds. The number of scans (8–256) and receiver gain were adjusted as needed for each sample. The reference for spin concentration was prepared from OF1. The polymer was dissolved in PBS (0.5 mM, pH 7.2) to provide 1.036 mM solution, for which concentration was calibrated with 3-carboxy-PROXYL in PBS buffer (0.5 mM, pH 7.2) at ambient temperature (295.0 K). This reference was always stored in dry ice, except during the measurement, and occasionally re-checked for spin concentration decay. How to cite this article: Sowers, M. A. et al. Redox-responsive branched-bottlebrush polymers for in vivo MRI and fluorescence imaging. Nat. Commun. 5:5460 doi: 10.1038/ncomms6460 (2014).